Pre-B cell receptor binding to galectin-1 modifies galectin-1/carbohydrate affinity to modulate specific galectin-1/glycan lattice interactions Galectins are glycan-binding proteins involved in various biological processes including cell/cell interactions. During B-cell development, bone marrow stromal cells secreting galectin-1 (GAL1) constitute a specific niche for pre-BII cells. Besides binding glycans, GAL1 is also a pre-B cell receptor (pre-BCR) ligand that induces receptor clustering, the first checkpoint of B-cell differentiation. The GAL1/pre-BCR interaction is the first example of a GAL1/unglycosylated protein interaction in the extracellular compartment. Here we show that GAL1/pre-BCR interaction modifies GAL1/glycan affinity and particularly inhibits binding to LacNAc containing epitopes. GAL1/pre-BCR interaction induces local conformational changes in the GAL1 carbohydrate-binding site generating a reduction in GAL1/glycan affinity. This fine tuning of GAL1/glycan interactions may be a strategic mechanism for allowing pre-BCR clustering and pre-BII cells departure from their niche. Altogether, our data suggest a novel mechanism for a cell to modify the equilibrium of the GAL1/glycan lattice involving GAL1/unglycosylated protein interactions. Lectins on cell surfaces mediate cell–cell contacts by interacting with specific carbohydrates on apposing cells. The lectins that bind to cell surface glycoproteins are often multivalent. As well, glycoproteins often bear multiple copies of the saccharide ligand that are recognized by lectins [1] , [2] . The multivalent nature of both lectins and their saccharide ligands allows the formation of a lectin–carbohydrate lattice, which acts as a signalling complex at the cell surface. These lectin–glycoprotein lattices are characterized by multiple low-affinity interactions, resulting in high overall avidity [3] , [4] , [5] . However, these organized interacting structures are not fixed and can be modified according to the cell’s needs. Only two modes have been described to dynamically modulate the strength of the lattice interactions: (i) altering protein glycosylation or (ii) altering lectin expression [6] . One family of multivalent lectins that can organize cell surface lattices is the galectins [7] . Galectins preferentially bind β-galactoside-containing glycans comprised of repeating units at the termini of complex N -glycans or as repeating units in a poly- N -acetyllactosamine chain on N -glycan or O -glycan [7] , [8] , [9] . The galectins share a common carbohydrate recognition domain (CRD) responsible for β-galactoside binding [10] and have been shown to be involved in cell interactions, proliferation, migration, apoptosis and mRNA splicing [3] , [11] , [12] , [13] . Galectins are also associated with different pathologies and most importantly with cancer [14] , thus providing targets for novel anticancer therapies. Among galectins, galectin-1 (GAL1) is differentially expressed by various normal and pathological tissues and appears to be functionally polyvalent, with a wide range of biological activities [15] . The overall folding of GAL1 involves a β sandwich consisting of two anti-parallel β-sheets forming a concave and a convex side. This jellyroll topology of the CRD constitutes the typical folding patterns of galectins. The concave side forms a groove which accommodates the carbohydrate: the carbohydrate-binding site (CBS). The CBS can be schematically described as having five subsites (A–E) with subsites C and D defining the conserved core β-galactoside-binding site [16] . Human GAL1 exists as a dimer in solution [17] and the presence of more than one CRD in a GAL1 homodimer makes it well suited for mediating cell adhesion, eliciting signalling and forming lattices [7] , [14] . We previously evidenced a crucial role of GAL1 in B-cell development through the formation of a GAL1-dependent lattice between pre-BII and stromal cells [18] , [19] , [20] , [21] . B cells are generated from haematopoietic stem cells and develop in the bone marrow before they migrate into the blood to reach peripheral lymphoid organs. While the diversity of B-cell repertoire is generated by the rearrangement of the Ig gene loci, checkpoints are needed during the differentiation process to ensure that the surface-expressed antigen-specific B-cell receptor (BCR) is functional yet not autoreactive [22] . Expression of the pre-B cell receptor (pre-BCR) represents a crucial checkpoint during B-cell development as this receptor controls pre-BII cell development and the selection of the Igμ repertoire [23] . We have found that pre-BII cells are associated to medullar stromal cells secreting GAL1 that constitute a specific pre-BII cell niche in the bone marrow [21] . At the contact zone between pre-BII and stromal cells, GAL1, pre-BCRs and glycosylated integrins relocalize [18] . This relocalization is allowed by the dual interaction network of GAL1 with the pre-BCRs (protein–protein interactions) and with glycosylated counter receptors (protein–oligosaccharide interactions) at the cell surfaces [18] , [19] , [20] . To date, this GAL1/pre-BCR interaction is the first example of a GAL1/unglycosylated protein interaction in the extracellular compartment. This immune ‘developmental synapse’ is accompanied by the initiation of intracellular tyrosine kinase activity and signal transduction from the pre-BCR [18] , [19] . The pre-BCR is constituted of two heavy chains, two surrogate light chains (SLCs) and the CD79a/b signalling molecules. GAL1 has been shown to interact directly to the SLC ( K D of 0.5 μM) (ref. 18 ). Each SLC is composed of the λ5 and VpreB proteins. The N terminus of λ5 and the C terminus of VpreB contain unique regions (λ5-UR and VpreB-UR, respectively) crucial for pre-BCR cell surface expression [24] , [25] and pre-BCR activation [18] , [24] . We recently found that GAL1 interacts with a λ5-UR motif, λ5-UR 22-45 , of the pre-BCR that adopts a stable helical conformation that docks onto a GAL1 hydrophobic surface adjacent to the CBS [26] . We hypothesized that this close proximity of the two interacting surfaces might then influence the carbohydrate-binding event when the λ5-UR 22-45 peptide is bound to GAL1. Interestingly, on λ5-UR binding, the lactose-binding activity of GAL1 undergoes a fourfold decrease, while no binding affinity changes have been observed for GAL1/λ5-UR 22-45 interaction in the presence versus in the absence of lactose [26] . These modulations suggest that the pre-BCR could modulate GAL1 affinity for specific glycoproteins [26] by a mechanism that would be a strategic step at the synapse level to modify the crosslinked lattices. Our hypothesis is supported by a recent study on a non-natural peptide, Anginex, suggesting that this peptide is able to enhance GAL1 carbohydrate-binding affinity for glycoproteins [27] . This peptide has been developed to inhibit tumour growth through specific inhibition of angiogenesis [28] , [29] . There are many text book cases where a stronger or weaker binding activity of one protein is induced by another protein or smaller molecule, but the molecular and structural basis of such effects have not been described yet for the carbohydrate-binding activity of galectins. Here we demonstrated that on binding to the λ5-UR of the pre-BCR, GAL1 undergoes selective affinity changes in its carbohydrate-binding activity. By exploring the glycome of pre-BII and stromal cells, we identified the presence of certain glycans for which GAL1 presents affinity changes when bound to the pre-BCR on the cell surfaces. These carbohydrate-binding activity changes have been explained at atomic resolution level by the modification of several intermolecular contacts between GAL1 and the carbohydrate. Such carbohydrate-binding modulation of GAL1 when bound to the pre-BCR allowed us to propose a model for the sequential interactions involved in pre-BCR relocalization and pre-BII cell departure from the niche. Collectively, our findings provide the structural basis of a new mechanism by which a galectin-dependent lattice can be dynamically modulated independently of alteration of protein glycosylation or lectin expression. Moreover, these results provide a new road map for developing inhibitors targeting galectin-dependent lattices in pathological situations such as cancers. GAL1 carbohydrate-binding specificity when bound to λ5-UR To investigate whether the changes induced by λ5-UR interaction to GAL1 modify its carbohydrate-binding specificity, we performed glycan array screenings of GAL1 free and bound to λ5-UR. Fluorescently labelled GAL1 at 5 μg ml −1 was used to probe a glycan array offered by the Consortium of Functional Glycomics (CFG; Fig. 1 ). GAL1 exhibits strong binding on glycan arrays toward LacNAc terminated complex type bi- and triantennary carbohydrates ( Supplementary Fig. 1 ) as it was previously observed [30] . The glycomic patterns for both GAL1 free and bound to λ5-UR, are similar ( Fig. 1a,b ) suggesting no drastic changes such as an on/off switch in binding specificity of GAL1 when bound to λ5-UR. However, the fluorescence intensities for several of these glycans are not strictly identical in the presence of λ5-UR. These changes were also observed when the same experiments were performed with GAL1 at 25 μg ml −1 ( Supplementary Fig. 2 ). Therefore, besides this global analysis, we performed a detailed cross-analysis of the two data sets by normalizing the relative fluorescence of each glycan on each array and compared if this normalized relative fluorescence has increased or decreased when λ5-UR is bound to GAL1 ( Fig. 1c ). The difference of normalized fluorescence intensities pinpoints changes in GAL1 binding for several glycans, when GAL1 is bound to λ5-UR ( Fig. 1c ). Increased binding of GAL1 is observed for structurally related groups of glycans including: (i) lactose and N -acetyllactosamine (LacNAc) mono or disulfated; (ii) α3 sialylLacNAc and α3 sialyllactotetraose glycans. In this study, we have considered and selected as significant only the carbohydrate-binding changes of the λ5-UR bound GAL1 when changes in structurally related groups of glycans are observed at 5 μg ml −1 ( Fig. 1 ) and 25 μg ml −1 ( Supplementary Fig. 2 ). We also observed significant decreased binding for several high binding glycans ( Supplementary Fig. 1 ) when GAL1 is bound to λ5-UR. Binding to three groups of structurally related glycans were then identified as decreased: (iii) branched LacNAc pentasaccharide; (iv) tetra- and hexasaccharides, mostly consisting of LacNac repeats fucosylated or not; (v) LacNAc complex type, biantennary carbohydrates fucosylated and unfucosylated. These data suggest that λ5-UR binding to GAL1 differentially modulates GAL1-binding activity for structurally related carbohydrates. 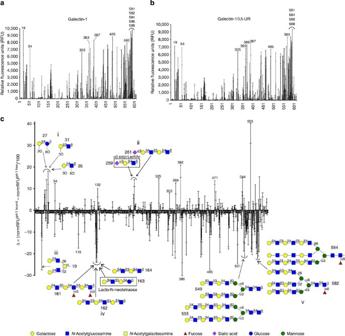Figure 1: Carbohydrate-binding specificity of GAL1 free and bound to λ5-UR. Fluorescently labelled GAL1 was analysed for binding to the mammalian glycan array (V5.1) of the CFG when free (a) or bound (b) to λ5-UR. Results shown for each plot are averages of two biological replicate measurements of fluorescence intensity at a lectin concentration of 5 μg ml−1. Error bars indicate the s.e.m. for two experiments. The raw data and the entire list of glycans with the respective spacers can be found on the CFG website (http://functionalglycomics.org/). Glycans presenting the highest relative fluorescence intensity are indicated with their number ID (The structure of these glycans is depicted inSupplementary Fig. 1). (c) Relative fluorescence intensity comparison for each glycan between free and λ5-UR bound GAL1. The fluorescence intensities measured inaandbhave been normalized and the differential plot between free and bound GAL1 has been generated. Positive and negative bars indicate a higher and a weaker binding of GAL1, respectively, for the glycan in the presence of λ5-UR. Glycan structures and number ID are depicted for several epitopes with significant relative fluorescence difference and sharing similar structural motifs (clusters of bars presenting significant differences are numbered from (i) to (v)). Figure 1: Carbohydrate-binding specificity of GAL1 free and bound to λ5-UR. Fluorescently labelled GAL1 was analysed for binding to the mammalian glycan array (V5.1) of the CFG when free ( a ) or bound ( b ) to λ5-UR. Results shown for each plot are averages of two biological replicate measurements of fluorescence intensity at a lectin concentration of 5 μg ml −1 . Error bars indicate the s.e.m. for two experiments. The raw data and the entire list of glycans with the respective spacers can be found on the CFG website ( http://functionalglycomics.org/ ). Glycans presenting the highest relative fluorescence intensity are indicated with their number ID (The structure of these glycans is depicted in Supplementary Fig. 1 ). ( c ) Relative fluorescence intensity comparison for each glycan between free and λ5-UR bound GAL1. The fluorescence intensities measured in a and b have been normalized and the differential plot between free and bound GAL1 has been generated. Positive and negative bars indicate a higher and a weaker binding of GAL1, respectively, for the glycan in the presence of λ5-UR. Glycan structures and number ID are depicted for several epitopes with significant relative fluorescence difference and sharing similar structural motifs (clusters of bars presenting significant differences are numbered from (i) to (v)). Full size image Quantification of GAL1 affinity changes for selected glycans To validate and quantify the changes observed on the glycan array data ( Fig. 1c ), we used isothermal titration calorimetry (ITC) measurements of GAL1 binding to selected glycans ( Supplementary Fig. 3 and Supplementary Table 1 ). We tested two glycans, the lacto- N -neotetraose (LNnT) belonging to group (iv) ( Fig. 1c ) and the α3 sialyl-N-Acetyllactosamine (α3 SiaLacNAc) belonging to group (ii) ( Fig. 1c ), for which a relative decrease and increase in GAL1 binding, respectively, are observed in the presence of the λ5-UR domain (binding of these two glycans to GAL1 has been demonstrated previously [31] , [32] ). In our experimental conditions, the dissociation constant ( K D ) of GAL1/LNnT interaction obtained is 51±6 μM, whereas when GAL1 is bound to the λ5-UR domain, the K D increases to 130±10 μM, that is, a 2.5-fold decrease in binding affinity of LNnT for GAL1 in the presence of λ5-UR ( Supplementary Table 1 ). The K D measured for GAL1/α3 SiaLacNAc complex formation is 240±20 μM. In the presence of λ5-UR, the K D reaches 25±2 μM, that is, a 10-fold increase in binding activity. As a control, we tested for binding the LacNAc for which no GAL1 binding change is observed in the presence of λ5-UR according to the glycan array. The K D evaluated from the ITC measurements do not show significant affinity changes when GAL1 is bound to λ5-UR ( Supplementary Table 1 ). Therefore, these results are in agreement with the binding changes of GAL1 for these glycans observed qualitatively on the glycan array screening ( Fig. 1c ). Altogether, the glycan array and ITC experiments demonstrate that λ5-UR binding to GAL1 is able to modify the GAL1 carbohydrate affinity for selected glycans. When placed in the context of the pre-B synapse, this phenomenon argues for pre-BCR-driven modification of the GAL1/glycans binding equilibria within the lattice. To investigate the presence on the cells forming the pre-B synapse of one or several groups of the identified glycans, it was then crucial to explore the glycome of pre-BII cells and stromal cells secreting GAL1 for which no glycomic data were available. Glycomic exploration of pre-BII and stromal cells GAL1 + To establish the biological relevance of the differences observed on glycan array screenings, we performed glycomic analysis of Nalm6 pre-BII and OP9 stromal cell lines using lectin microarray experiments. These cell lines have been chosen since they have been used in many functional assays [18] , [19] , [20] , [26] to study the role of GAL1 and GAL1/pre-BCR interaction for pre-BCR relocalization and signalling. We have shown previously that, similarly to normal pre-BII cells, the Nalm6 pre-B cell line expresses pre-BCRs and integrins required for the formation of the pre-B cell synapse and the induction of an efficient pre-BCR signal [18] , [19] , [20] , [26] . In addition, OP9 stromal cells were shown to strongly support normal pre-BII cell differentiation, due to the expression of GAL1 and integrin ligands required for the formation of the pre-B cell synapse [20] . Therefore, even though immortalized cells often show alterations of cell surface receptors, pre-BCR relocalization and signalling using Nalm6 and OP9 cells reflect what is observed in primary cells. 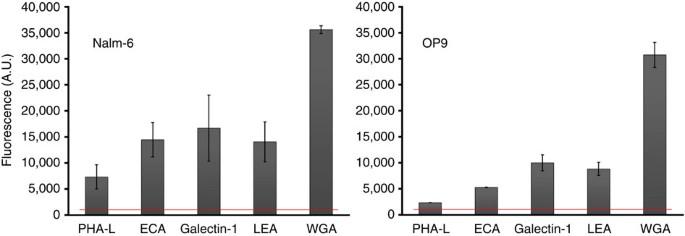Figure 2: Nalm6 pre-BII and OP9 stromal cells contain GAL1 ligands. Single-colour analysis of poly/multiantennary LacNAc on OP9 and Nalm6 by lectin microarray is shown. Graph displays the median normalized fluorescence for selected LacNAc binding lectins binding to OP9 and Nalm6. All lectins are above the 1,000 fluorescence unit threshold for binding (red line) and show signal-to-noise ratios >5, defining them as positive. Error bars represent s.d. forn=3 spots on a single microrarray. These data are consistent with previous results on a biological replicate. Binding of lectin is as follows: GAL1, Galectin-1 ligands; LEA, polyLacNAc chains; PHA-L: multiantennary LacNAc, WGA and ECA: terminal LacNAc residues. In lectin microarrays, carbohydrate-binding proteins (lectins; for a list of lectin abbreviations, see Supplementary Table 2 ) are immobilized onto a solid support at a high spatial density [33] , [34] . Interrogation of the arrays with fluorescently labelled sample enables elucidation of the glycome based on the distinct carbohydrate-binding specificities of the lectins. This method has been used to analyse the glycomic fingerprint of viruses [35] , bacteria [36] , mammalian cells [37] and tissues [38] in a high-throughput manner. Profiling of Nalm6 pre-BII and OP9 stromal cell samples using single-colour analysis showed that both cell types displayed GAL1 ligands such as poly/multiantennary LacNAc as confirmed by GAL1, ECA, LEA, PHA-L and WGA binding on the arrays ( Fig. 2 ; for a list of lectin abbreviations, see Supplementary Table 2 ). More specific epitopes such as α3 sialylated/sulfated glycans as well as bi-and multiantennary N -glycans are found on both cell types thus indicating the presence of group (i) to (v) glycan epitopes on both cells ( Fig. 3 ). Given that the stromal cells have high secretion of GAL1, it was important to address if this lectin could occlude binding of the galectin ligands by the lectins on the microarray. To address this concern, cells were treated with lactose. Cells treated with lactose showed no significant differences in glycan signature compared with untreated OP9 ( Supplementary Fig. 4 ), indicating that sample preparation before hybridization on the array (cell sonication and extensive dialysis) [37] remove most of the GAL1 bound to the cells. Figure 2: Nalm6 pre-BII and OP9 stromal cells contain GAL1 ligands. Single-colour analysis of poly/multiantennary LacNAc on OP9 and Nalm6 by lectin microarray is shown. Graph displays the median normalized fluorescence for selected LacNAc binding lectins binding to OP9 and Nalm6. All lectins are above the 1,000 fluorescence unit threshold for binding (red line) and show signal-to-noise ratios >5, defining them as positive. Error bars represent s.d. for n =3 spots on a single microrarray. These data are consistent with previous results on a biological replicate. Binding of lectin is as follows: GAL1, Galectin-1 ligands; LEA, polyLacNAc chains; PHA-L: multiantennary LacNAc, WGA and ECA: terminal LacNAc residues. 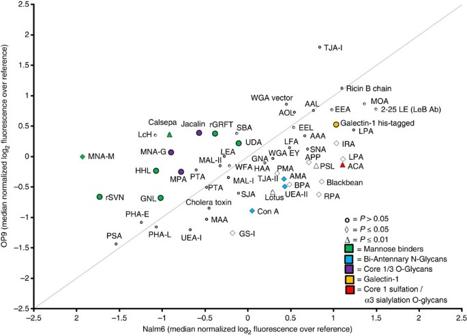Figure 3: Glycosylation differences for Nalm6 pre-BII versus OP9 stromal cells as identified using dual-colour lectin microarrays experiments. Biplot of lectin array data averaged over three biological replicates for Nalm6 versus OP9 cells. Colour represents lectin binding preference and shape represents levels ofPbased on Student’st-test. Full size image Figure 3: Glycosylation differences for Nalm6 pre-BII versus OP9 stromal cells as identified using dual-colour lectin microarrays experiments. Biplot of lectin array data averaged over three biological replicates for Nalm6 versus OP9 cells. Colour represents lectin binding preference and shape represents levels of P based on Student’s t -test. Full size image To identify the higher expression of one or several glycans on one of the cell type with respect to the other, biological triplicates of Nalm6 pre-BII and OP9 stromal cell samples were analysed using dual-colour lectin microarray technology, which provides a more sensitive and semi-quantitative comparison [37] . This analysis revealed no significant differences in poly/multiantennary LacNAc levels, although specific glycomic profiles for each cell type were observed ( Fig. 3 ). OP9 Stromal cells were significantly enriched in high mannose ( Fig. 3 , Calsepa, GNL, HHL, MNA-M, rGRFT rSVN, UDA, P <0.05 for Calsepa and MNA-M, Student’s t -test). Core 1/3 O -glycans were also enriched, although individually none of the lectins were significantly so (Jacalin, MNA-G, MPA). Pre-BII cells showed significant enrichment in biantennary N- glycans (AMA ConA, UEA-II, P <0.05 for all three lectins) and in binding to α3 sialylated/sulfated core-1 O -glycans (ACA, P <0.01, for annotation see CFG data set, [39] ). These experiments suggest that biantennary N- glycans found in group (v) ( Fig. 1c ) and α3 sialylated/sulfated core-1 O -glycans, whose groups (i) and (ii) glycan epitopes can be part of ( Fig. 1c ), are more exposed on Pre-BII cells compared with stromal cell lines. Our glycan and lectin array experiments indicate that, when bound to the pre-BCR, GAL1 would modify its glycan-binding equilibria within the synapse by changing its affinity for glycans found on both cell types inducing a fine tuning of the lattice interactions at the synapse level. To understand at the atomic level how these variations in GAL1 carbohydrate binding can occur, a more detailed structural analysis of GAL1 carbohydrate binding in the presence of λ5-UR is needed. The GAL1/LNnT and GAL1-λ5-UR 22-45 /LNnT interactions To elucidate the structural basis of the consequences induced by λ5-UR binding on carbohydrate activity of GAL1, we have further studied GAL1 interaction with the Lacto- N -neotetraose (group (iv), Fig. 1c ), motif which can be part of a more complex glycan structure at the cell surface, using ITC and NMR spectroscopy. For this structural study, we used the λ5-UR 22-45 peptide, a 24 amino-acid peptide of the λ5-UR domain shown to be sufficient for interaction with GAL1 (ref. 26 ). We first checked using ITC that the presence of the λ5-UR 22-45 peptide induces the same GAL1 affinity changes for LNnT as the full-length λ5-UR domain does. Indeed, a threefold decrease in binding affinity is observed when GAL1 is complexed to the λ5-UR 22-45 peptide ( Supplementary Table 1 and Supplementary Fig. 5 ) as similarly shown above when GAL1 is complexed to the full-length λ5-UR domain ( Supplementary Table 1 and Supplementary Fig. 3a,b ). We then mapped the interaction sites of LNnT on GAL1 using NMR spectroscopy ( Figs 4 and 5 , respectively). We first monitored the NMR resonances of the 15 N-labelled GAL1 in the absence and in the presence of LNnT ( Fig. 4a ). Addition of LNnT elicited large chemical shift perturbations (CSPs) in a subset of 15 N-labelled GAL1 amide resonances. A single cross-peak per GAL1 amide was observed during the titration, indicating a fast exchange between the free and the bound states on the NMR timescale, in accordance with the K D observed using ITC (110 μM). As expected, most of the perturbations co-localize mainly to the CBS ( Fig. 4b ) including residues His52, Trp68, Arg73 and Val59 which are known to provide stacking Van Der Waals interactions or hydrogen bonds with carbohydrates. The residues undergoing significant chemical shift variations belong to the subsite C (Asn50, His52, Trp68), D (Gly53, Asp54, val59, Glu71, Arg73) and E (Gly69, Thr70) of the CBS [16] . It is to be noticed that the subsite D is directly adjacent to the λ5-UR 22-45 -interacting surface. Few residues from the backside of the protein, including Cys16, Phe91 and Gly103, were also significantly perturbed. It has been previously observed in the case of lactose binding to 15 N-labelled GAL1 that similar CSPs are induced, that is, at and away from the GAL1 CBS, suggesting that conformational dynamic perturbations could occur in the protein on carbohydrate binding [40] . 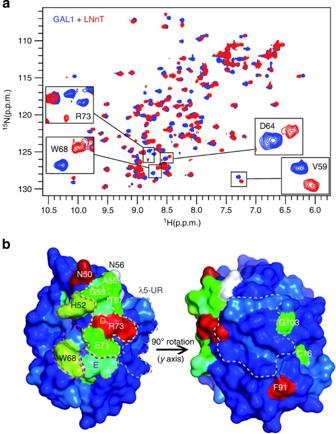Figure 4: Mapping LNnT binding on GAL1. (a) Overlay of 2D1H,15N HSQC spectra of GAL1 in the free form (blue) and with a fourfold molar excess of LNnT (red). Expanded regions show resonances representative of those that showed large CSPs on binding to LNnT. (b) CSPs induced by LNnT binding mapped onto the GAL1 surface (PDB 1GZW). Monomer surface structure is represented. CSPs have been coloured from blue to iodine (CSP<0.05: blue, <0.1 marine, <0.125: greencyan, <0.15: green, <0.175: lemon, <0.2: yellow orange, <0.225: orange, <0.25: red, <0.275: iodine). White is used for unassigned residue resonances. Subsites C–E of the GAL1 CBS are delineated with pink and yellow dotted lines. The λ5-UR22-45-interacting site is indicated using dotted grey lines. Figure 4: Mapping LNnT binding on GAL1. ( a ) Overlay of 2D 1 H, 15 N HSQC spectra of GAL1 in the free form (blue) and with a fourfold molar excess of LNnT (red). Expanded regions show resonances representative of those that showed large CSPs on binding to LNnT. ( b ) CSPs induced by LNnT binding mapped onto the GAL1 surface (PDB 1GZW). Monomer surface structure is represented. CSPs have been coloured from blue to iodine (CSP<0.05: blue, <0.1 marine, <0.125: greencyan, <0.15: green, <0.175: lemon, <0.2: yellow orange, <0.225: orange, <0.25: red, <0.275: iodine). White is used for unassigned residue resonances. Subsites C–E of the GAL1 CBS are delineated with pink and yellow dotted lines. The λ5-UR 22-45 -interacting site is indicated using dotted grey lines. 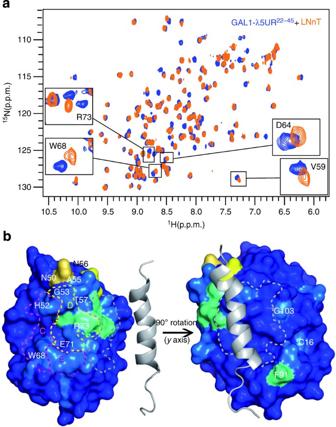Figure 5: Mapping LNnT binding on GAL1 in the presence of the λ5-UR22-45peptide. (a) Overlay of 2D1H,15N HSQC spectra of GAL1 bound to λ5-UR22-45(blue) and with a fourfold molar excess of LNnT (orange). Expanded regions show resonances representative of those that showed large CSPs on binding to LNnT. (b) CSPs induced by LNnT binding mapped onto the GAL1 surface (PDB 1GZW). Monomer surface structure is represented. CSPs have been coloured from blue to iodine (CSP<0.05: blue, <0.1 marine, <0.125: greencyan, <0.15: green, <0.175: lemon, <0.2: yelloworange, <0.225: orange, <0.25: red, <0.275: iodine). White is used for unassigned residue resonances. Subsites C–E of the GAL1 CBS are delineated with pink and yellow dotted lines. The λ5-UR22-45peptide is represented as grey ribbon and its interacting surface on GAL1 is delineated with dotted lines. Full size image Figure 5: Mapping LNnT binding on GAL1 in the presence of the λ5-UR 22-45 peptide. ( a ) Overlay of 2D 1 H, 15 N HSQC spectra of GAL1 bound to λ5-UR 22-45 (blue) and with a fourfold molar excess of LNnT (orange). Expanded regions show resonances representative of those that showed large CSPs on binding to LNnT. ( b ) CSPs induced by LNnT binding mapped onto the GAL1 surface (PDB 1GZW). Monomer surface structure is represented. CSPs have been coloured from blue to iodine (CSP<0.05: blue, <0.1 marine, <0.125: greencyan, <0.15: green, <0.175: lemon, <0.2: yelloworange, <0.225: orange, <0.25: red, <0.275: iodine). White is used for unassigned residue resonances. Subsites C–E of the GAL1 CBS are delineated with pink and yellow dotted lines. The λ5-UR 22-45 peptide is represented as grey ribbon and its interacting surface on GAL1 is delineated with dotted lines. Full size image We next performed the same NMR experiments with a preincubation of GAL1 with λ5-UR 22-45 peptide to allow the protein–peptide complex formation. Titrations of LNnT to the 15 N-GAL1/λ5-UR 22-45 complex showed weaker GAL1 resonance perturbations indicative of a weaker binding of the carbohydrate when GAL1 is complexed to the peptide ( Fig. 5 and Supplementary Fig. 6 ). This result is in agreement with the observed K D and glycan array experiments. Among the perturbed resonances, Arg73 showed the strongest decrease in chemical shift variations when GAL1 is bound to the peptide ( Fig. 5b and Supplementary Fig. 6 ). Arg73 belongs to subsite D of the CBS and is really localized at the junction between the CBS and the λ5-UR-binding site ( Fig. 5b ). Analysis of the structure of the GAL1/λ5-UR 22-45 complex [26] shows that Arg73 is oriented toward the peptide in the GAL1 bound conformation, whereas it faces the CBS and therefore the carbohydrate in the peptide free conformation of GAL1 ( Fig. 6 ). Altogether our data suggest that binding of the λ5-UR 22-45 peptide to GAL1 induces structural modifications in the subsite D of the CBS among which Arg73 side-chain reorientation. These changes lead to carbohydrate binding destabilization resulting in the observed reduced affinity of GAL1 for LNnT. 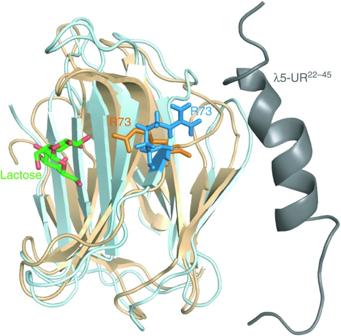Figure 6: Structural changes induced by λ5-UR22-45binding to GAL1. The structures of GAL1/λ5-UR22-45(in light blue and grey, respectively) and GAL1/lactose17(in beige and green, respectively) complexes are superimposed. Side chains of Arg73 residue from each structure are represented and labelled. Figure 6: Structural changes induced by λ5-UR 22-45 binding to GAL1. The structures of GAL1/λ5-UR 22-45 (in light blue and grey, respectively) and GAL1/lactose [17] (in beige and green, respectively) complexes are superimposed. Side chains of Arg73 residue from each structure are represented and labelled. Full size image Epitope mapping of LNnT bound to GAL1 and GAL1/λ5-UR 22-45 Since λ5-UR binding to GAL1 induces structural modifications resulting in a binding affinity decrease of GAL1 for LNnT, we next investigated at atomic resolution the mode and orientation of LNnT binding to GAL1 and GAL1/λ5-UR using saturation transfer difference (STD) NMR experiments [41] ( Fig. 7 ). STD-NMR is a ligand-based NMR experiment enabling the mapping of the ligand’s binding epitope. The STD NMR protocol is based on the intermolecular saturation transfer from the protein to the binding part of the ligand. The part of the ligand having the strongest contact to the protein shows the most intense NMR signals. As a first step to this study, we assigned 13 C (96%) and 1 H (100%) NMR resonances of LNnT using homo- and heteronuclear two-dimensional (2D) NMR experiments ( Fig. 7a ). STD-NMR experiments were recorded on a sample containing a 100-fold molar excess of LNnT relative to GAL1 before and after addition of threefold molar excess of λ5-UR 22-45 . Some characteristic features of the LNnT-binding epitope are revealed by the inspection of 1D STD-NMR spectra. In the presence of GAL1 ( Supplementary Fig. 7 ), a clear binding epitope exists since not all of the 1 H NMR signals of the tetrasaccharide ( Supplementary Fig. 7 ) were displayed in the STD spectrum. The N -acetyl group attached to the N -acetylglucosamine (HN GlcNAc ), and the H1 and H4 from the internal galactose (C) moiety clearly receive strong saturation transfer, whereas the H1 and H2 from the glucose (D) moiety receive much less. Therefore, these spectra suggest that the GlcNAc and the internal galactose residues are in close proximity with GAL1. When the λ5-UR peptide is bound to GAL1 ( Supplementary Fig. 7 ), the STD spectrum is globally similar to the one recorded in the absence of λ5-UR 22-45 ( Supplementary Fig. 7 ) but significant differences in peak intensities can be observed especially in the 4.0 to 3.4 p.p.m. region. At this stage, due to heavy overlapping observed in this region, no fine details of the contributing moieties could be obtained in an unambiguous manner. To obtain information on ligand signals that are heavily overlapped, 2D STD TOCSY experiments were performed to resolve the STD signal in a second dimension ( Fig. 7 ). A simple epitope mapping on the basis of STD TOCSY spectra is easily achieved for isolated spin systems, such as the ones found for pyranose rings in oligosaccharides. Spin diffusion across glycosidic linkages can be neglected and, therefore, a qualitative comparison of the corresponding cross-peaks readily identifies pyranose units in intimate contact with the GAL1 CBS. It is immediately obvious that mainly the cross-peaks of the GlcNAc (B) display the largest overall intensities ( Fig. 7b ), indicating that the protons of this pyranose ring are in close contact with the GAL1 protein as suggested in the 1D STD spectrum ( Supplementary Fig. 7 ). The internal galactose (C) and the glucose (D) moieties present significant cross peak intensities thus indicative of proximity with the protein. The terminal galactose (A) provided few and weaker STD effects indicating that it mainly remains outside of the main protein-binding site. Relative ranking of the amount of saturation that is transferred to individual spin have been done for LNnT binding to GAL1 ( Fig. 7b , right panel). The major contributions for GAL1/LNnT binding involve H2, H4 and H6 from the GlcNAc (B) moiety, H1 and H4 from the internal Gal (C), and H3 and H4 from the terminal glucose (D). When GAL1 is bound to the λ5-UR 22-45 peptide, several cross-peaks of the STD spectrum show a significant global decrease of STD signals ( Fig. 7c ). These observations are indicative of a loss of several LNnT/GAL1 contacts in the presence of the λ5-UR peptide. Integration of 2D STD signals revealed that the contacts involving H3 and H4 from the terminal glucose (D) experienced the strongest decrease in STD signal intensity ( Fig. 7c , right panel). Indeed, while most of the STD signals are decreased by 35% on average, the STD signals from H3 and H4 from the terminal glucose decrease by ~70%. These results indicate that the λ5-UR peptide induces a loss of contacts mainly at the level of the terminal glucose (D) thus affecting the strength of binding of the rest of the LNnT molecule. 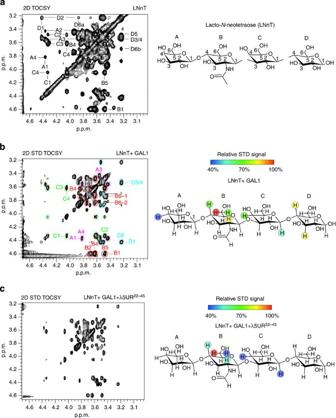Figure 7: Mapping the LNnT-binding epitope using 2D STD-NMR spectroscopy. (a) 2D TOCSY spectrum of LNnT (from 3.1 to 4.6 p.p.m.) is shown on the left panel with several cross-peaks assignment. Proton cross-peaks are labelled according to the nomenclature shown on the right panel. (b) 2D STD TOCSY spectrum of LNnT in the presence of GAL1 is represented on the left panel. The cross-peaks showing the highest intensity are circled and assignment is indicated. The circles are colour coded according to the monosaccharide they belong to: terminal galactose: magenta,N-acetylglucosamine: red, internal galactose: green, terminal glucose: blue. On the right panel, the significant relative STD signals observed are reported on the LNnT and are colour coded according to the colour scale shown above. The 100% STD signal corresponds to the resonance showing the highest intensity contribution in each experiment; all other STD signals are calculated accordingly. (c) 2D STD TOCSY of LNnT+GAL1+λ5-UR22-45is shown on the left panel. On the right panel, the relative STD signals observed are reported on the LNnT as inb. Figure 7: Mapping the LNnT-binding epitope using 2D STD-NMR spectroscopy. ( a ) 2D TOCSY spectrum of LNnT (from 3.1 to 4.6 p.p.m.) is shown on the left panel with several cross-peaks assignment. Proton cross-peaks are labelled according to the nomenclature shown on the right panel. ( b ) 2D STD TOCSY spectrum of LNnT in the presence of GAL1 is represented on the left panel. The cross-peaks showing the highest intensity are circled and assignment is indicated. The circles are colour coded according to the monosaccharide they belong to: terminal galactose: magenta, N -acetylglucosamine: red, internal galactose: green, terminal glucose: blue. On the right panel, the significant relative STD signals observed are reported on the LNnT and are colour coded according to the colour scale shown above. The 100% STD signal corresponds to the resonance showing the highest intensity contribution in each experiment; all other STD signals are calculated accordingly. ( c ) 2D STD TOCSY of LNnT+GAL1+λ5-UR 22-45 is shown on the left panel. On the right panel, the relative STD signals observed are reported on the LNnT as in b . Full size image When compiled together, the results obtained on GAL1 binding to LNnT using ITC and NMR support a structural modification of the CBS when the λ5-UR peptide is bound to GAL1. Indeed, an unfavourable entropy is observed ( Supplementary Table 1 ) that could indicate a decrease of flexibility in the CBS on λ5 binding thus changing the CBS dynamic properties for LNnT binding. In that sense, we previously observed that binding of the λ5-UR peptide to GAL1 induces NMR CSPs on the backside of the protein, its interacting surface, but also in the subsites C and D of the CBS [26] . Accordingly, we can propose that the GlcNAc and the internal galactose of LNnT bind to the center of the CBS subsites C and D of GAL1, whereas the terminal glucose is localized in the part of the subsite D of the CBS that undergoes structural rearrangements on λ5-UR binding, as illustrated by Arg73 side-chain reorientation. This structural change leads to a loss of contacts between LNnT and GAL1 and thus a decrease of GAL1/LNnT affinity. We can therefore conclude that GAL1/λ5-UR interaction inhibits GAL1/LNnT binding as suggested by glycan array experiments ( Fig. 1c ). Galectin/glycan lattices play leading roles in signal transduction in different biological processes as well as in cell–cell interactions [42] . To the best of our knowledge, the GAL1/pre-BCR interaction is the first example of a GAL1/protein interaction with an unglycosylated protein-binding partner (λ5−UR) in the extracellular compartment. We have demonstrated that λ5-UR binding to GAL1 induces structural modifications in the CBS including Arg73 side-chain reorientation ( Fig. 6 ) probably associated to a decrease in CBS flexibility. Indeed, GAL1/λ5-UR complex formation leads to CSPs throughout the CBS from subsite A to E [26] . LNnT, a glycan that represents group (iv) as designated in Fig. 1c , binds mainly to subsites C to E of the GAL1 CBS ( Fig. 4 ). Together with groups (iii) and (v), these structures show a weaker binding to GAL1 bound to λ5-UR. Groups (iii) and (v) present branched and/or more extended structures compared with the LNnT that would protrude from the D subsite of GAL1 towards subsite E and towards the λ5-UR-binding site. Therefore, one can expect that the CBS modifications induced by the λ5-UR interaction to GAL1 perturb the binding of these glycans as suggested by the glycan array data ( Fig. 1c ). Conversely, glycans from groups (i) and (ii) among which α3 SiaLacNAc, showing enhanced binding to GAL1 when complexed to λ5-UR ( Fig. 1c , Supplementary Fig. 3c,d and Supplementary Table 1 ), contain sulfate groups or α3 sialylation on the terminal galactose. These sugar modifications should be localized at the subsites A–B for galactose modifications and at subsite D’ (top of subsite D) for Lac or GlcNAc modifications as suggested previously [30] . This localization is no within the structurally negative perturbations induced by λ5-UR binding evidenced at the subsite D ( Figs 5 , 6 , 7 ), explaining the differential effects of λ5-UR binding on recognition of groups (i) and (ii) versus groups (iii) to (v) as seen on the glycan arrays ( Fig. 1c ). Studies on the non-natural peptide anginex have shown that it greatly enhances the affinity of GAL1 for certain ligands, including biologically relevant glycoproteins [27] . Moreover, a topomimetic of anginex, the calixarene 0118, has been shown to be an allosteric inhibitor of GAL1 lactose binding, interacting with a surface of GAL1 located on the back face of the protein [43] . Therefore, anginex have opposite effects on GAL1 carbohydrate-binding activity depending on the carbohydrate substrate tested. Here we observed a threefold decrease for LNnT and a 10-fold increase for α3 SiaLacNAc GAL1-binding affinity in the presence of λ5-UR. We cannot exclude that λ5-UR could induce a higher effect on GAL1 binding to other more complex glycans and entire glycoproteins. It has been proposed that anginex may mimic a normal function, meaning that there is a natural counterpart in vivo [27] . Therefore, unglycosylated protein binding to GAL1 could represent a key regulator of GAL1/glycan interactions in the extracellular compartment. Relative concentration of GAL1 and of its various ligands can change the affinities within the crosslinked GAL1-dependent lattices. In that sense, dynamic modulation by the cell of protein glycosylation or lectin expression at the cell surface has been proposed as ways for the cell to modify its lectin/glycan equilibria. Quantification of the affinity change with the LNnT led to a threefold decrease in GAL1/LNnT-binding affinity in the presence of λ5-UR. A 10-fold increase in GAL1 binding has been observed for α3 SiaLacNAc. A three- or a 10-fold change on these individual interactions will result in a more dramatic effect within the context of galectin/glycan lattices consisting of multivalent interactions generating high avidity. Indeed, calixarene 0118 has been shown to be a potent angiogenesis inhibitor in vitro , as determined by endothelial cell proliferation, migration and chick embryo chorioallantoic membrane assays [44] and was also found to be highly effective at inhibiting tumour angiogenesis and tumour growth in murine tumour models (that is, MA148 human ovarian carcinoma and B16 murine melanoma) [44] . This molecule targets GAL1 as does Anginex at a site away from the CBS and attenuates lactose binding to the lectin by a threefold [43] illustrating that a threefold difference in affinity can be relevant to an in vivo situation. This process is not an on/off switch of GAL1 carbohydrate specificity; rather, we conclude that there is a fine tuning of the affinity of these interactions depending on the cell needs. This is an original and unforeseen way for a cell to modify the equilibria of the GAL1/glycan lattice besides changes in protein glycosylation or lectin expression. To shed light on the in vivo situation, modulation of GAL1 binding at the surface of OP9 stromal cells in presence or in absence of λ5-UR has been investigated by flow cytometry. No significant variations have been observed (data not shown). It has been shown that GAL1 is involved in different processes through the interaction with several glycans expressed by multiple proteins [7] . As a consequence, a large amount of GAL1 is found associated to the stromal cell membrane even without the formation of a synapse with a pre-B cell [18] . We have shown in the current work that lots of the glycans do not undergo GAL1 affinity changes ( Fig. 1c ). We therefore believe that affinity changes with GAL1 would only be induced for glycans involved in pre-BCR clustering, but not for the glycans expressed by proteins unrelated to that process. This would mean that it would be possible to target specifically one among several GAL1 cellular functions through a GAL1/unglycosylated protein interaction. The use of lectin microarrays allowed us to investigate the glycome of Nalm6 pre-BII and OP9 stromal cells. Lectins have been used for decades to elucidate glycan structure and our latest mapping of their specificities with the glycan arrays of the CFG (see online data sets on CFG website and ref. 39 ) has given us an ability to clearly identify structures from our data sets especially when using multiple lectins in combination. The glycomic exploration of the pre-BII cells and stromal cells secreting GAL1 highlighted the presence of LacNAc epitopes at the pre-BII and stromal cell surfaces ( Fig. 2 ) as well as a clear biantennary N -glycans and sulfated/α3 sialylated glycan signatures on pre-BII cells ( Fig. 3 ). The presence of GAL1 ligands on both cell types supports the crucial role of GAL1 in pre-BII/stromal cell recognition within the pre-BII cell niche. Indeed, it has been shown that pre-BII cells are not able to contact stromal cells that are not secreting GAL1 (ref. 21 ). The significant LacNAc content of pre-BII cells is therefore an important determinant for cell recognition and cell niche specificity. Our glycome analysis combined to the structural and affinity modifications observed on GAL1 when bound to λ5-UR indicates that the GAL1/glycan lattice at the pre-B synapse is modified to the disadvantage of glycans present on both cells (polyLacNAc) but in the advantage of epitopes found preferentially on pre-BII cells (sulfated/α3 sialylated glycans). Currently, the model of synapse formation [18] , [19] starts with the binding of stromal cell-derived GAL1 to pre-B cell glycosylated integrins and directly to the pre-BCR. Then, active integrin relocalization in the presence of GAL1 drives the pre-BCRs, through GAL1/pre-BCR interaction, into the pre-B/stromal cell synapse, leading to the initiation of pre-BCR signalling [19] . Our results complete this model ( Fig. 8 ). Once exposed at the surface of the stromal cells, GAL1 is associated with stromal glycosylated receptors containing LacNAc epitopes ( Fig. 8a ). When the pre-BII cell contacts the stromal cell through the interaction between pre-BII cell integrins and their ligands on stromal cells (fibronectin and ADAM-15, as previously identified [19] ), GAL1 is able to interact with the pre-BCR ( Fig. 8b ). We have shown that this interaction weakens the strength of GAL1 binding to LacNAc epitopes, that is, to glycan motifs present on both cells. GAL1 bound to pre-BCR might then be able to interact with other glycan motifs ( Fig. 8c ) such as α3 SiaLacNAc (group (ii), Fig. 1c ) found preferentially on pre-BII cells ( Fig. 3 ). GAL1 acts as the molecular link between pre-BCRs and relocalizing integrins leading the pre-BCRs into the synapse where they are then activated ( Fig. 8d ). The reduced affinity of GAL1 for stromal cell ligands should thus help the pre-BCRs internalization by endocytosis which takes place after pre-BCR activation. Moreover, this dissociation should participate significantly to the release of the pre-B cells from the niche, thus allowing the cells to migrate toward a new niche corresponding to another differentiation stage [45] . This spatial and temporal reorganization of the lattice would have direct consequences on synapse formation and dissolution. These interaction models are appealing as they help to explain how GAL1 can modify its lattice equilibria to form cell/cell contacts within a niche and subsequently modulate these contacts to allow cell departure from the niche. These findings may be extrapolated to other haematopoietic cell niches where there is increasing evidence that galectin–glycan interactions control communication between haematopoietic and non-haematopoietic cells [46] . 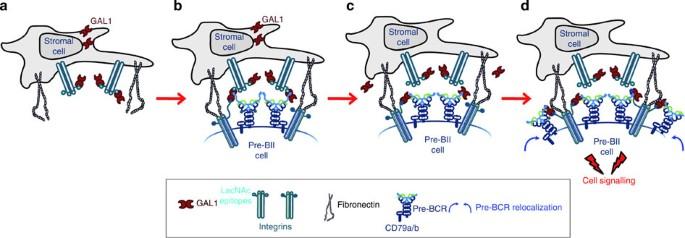Figure 8: Model of pre-B cell synapse formation. (a) GAL1 secreted by stromal cells is bound to LacNAc epitopes presented by stromal cell integrins and receptors. (b) When a pre-BII cell contacts the stromal cell, pre-BII cell integrins interact with their stromal cell ligands and GAL1 can bind Pre-BCRs and glycosylated receptors. (c) On binding to the pre-BCRs, GAL1 undergoes a decreased affinity for LacNAc epitopes thus weakening its anchoring to both cell glycans. GAL1 is then available for interaction to better ligands found on pre-BII cell relocalizing integrins. (d) The molecular link established by GAL1 between relocalizing pre-BII cell integrins and pre-BCRs drives these latters at the contact zone between the two cells. Relocalization of the pre-BCRs leads to cell signalling necessary for pre-BII cell differenciation and proliferation. Figure 8: Model of pre-B cell synapse formation. ( a ) GAL1 secreted by stromal cells is bound to LacNAc epitopes presented by stromal cell integrins and receptors. ( b ) When a pre-BII cell contacts the stromal cell, pre-BII cell integrins interact with their stromal cell ligands and GAL1 can bind Pre-BCRs and glycosylated receptors. ( c ) On binding to the pre-BCRs, GAL1 undergoes a decreased affinity for LacNAc epitopes thus weakening its anchoring to both cell glycans. GAL1 is then available for interaction to better ligands found on pre-BII cell relocalizing integrins. ( d ) The molecular link established by GAL1 between relocalizing pre-BII cell integrins and pre-BCRs drives these latters at the contact zone between the two cells. Relocalization of the pre-BCRs leads to cell signalling necessary for pre-BII cell differenciation and proliferation. Full size image More generally, GAL/glycan lattices include many pharmaceutically relevant targets that cover biologically important processes, such as proliferation, migration or apoptosis [7] , [47] . In this regard, galectin inhibitors that block the CRD have been developed for cancer treatment [48] , [49] , [50] . Although promising, several of these inhibitors lack selectivity for individual members of the galectin family and often display weak ligand affinities. In this study, we provided the structural basis of a GAL1/glycan inhibition through the GAL1/λ5-UR interaction. Our results provide the structural proof that it is possible to selectively inhibit GAL1/glycan interactions at distance of the CBS. Consequently, our results can be exploited for destabilization of GAL1/glycan interactions involved in cancers and will affect the development and design of new GAL1 inhibitors through GAL1/protein interactions. Protein preparation Plasmid encoding the human λ5-UR domain was used [26] to produce an amino-terminal His 6 tag domain fused to a lipoyl sequence (17), followed by a tobacco etch virus cleavage site. For the purification of the λ5-UR, the cells were disrupted using a French press, and the resulting supernatant was clarified by centrifugation at 125,000 g . The clarified supernatant was applied to a 5- ml HisTrap HP column (GE Healthcare, Piscataway, NJ) in accordance with the manufacturer’s instructions. After elution, the lipoyl domain was removed from the λ5-UR by tobacco etch virus protease digestion. The digestion mixture was applied to a HisTrap HP column. The flow-through containing the cleaved λ5-UR was concentrated in an Amicon (Millipore) concentrator, and the samples were applied to a Superdex 75 (10/300GL) gel filtration column (GE Healthcare) as a final purification step. For ITC experiments, the gene encoding human GAL1 was cloned into pET28a plasmid to produce a protein with a His 6 amino-terminal tag. After transformation of BL21(DE3) competent cells with the latter plasmid, bacteria were grown at 37 °C until OD 600 nm =0.6 then 1 mM isopropyl-β- D -thiogalactoside was added to the culture to start overexpression of the protein. After 4 h incubation at 37 °C, cells are harvested by centrifugation (3,000 g , 15 min). After cell lysis, the His 6 -tagged GAL1 is purified from the supernatant by affinity chromatography using HiTrap 5 ml prepacked column plugged to an AKTAPrime purifying system. Protein is eluted using a linear gradient of imidazole and then loaded onto a gel filtration column for further purification. For NMR experiments, 15 N-labelled GAL1 has been produced by growing the transformed cells in M9 minimal medium supplemented with 1 g l −1 15 NH 4 Cl (ref. 26 ). Protein purity is checked by Coomassie blue staining of a SDS–polyacrylamide gel electrophoresis. Peptide The λ5-UR 22-45 peptide used in the ITC and NMR experiments was chemically synthesized and purchased (Schafer-N, Copenhagen, Denmark). Carbohydrates The chemically synthesized LNnT was offered by Core D of the Consortium for Functional Glycomics (CFG). α3 SiaLacNAc was purchased from ELICITYL company. Glycan array screening Purified GAL1 was fluorescently labelled with Alexa Fluor 488 (Invitrogen) according to the manufacturer’s protocol and used (at a final concentration of 5 μg ml −1 in the absence and in the presence of two molar excess of λ5-UR) to probe versions 5.1 of the mammalian glycan array offered by Core H of the Consortium for Functional Glycomics (CFG). Each experiment has been performed on two biological replicates. The same experiments have been also performed at 25 μg ml −1 GAL1 concentration. For fluorescence intensity comparison for each glycan between free and λ5-UR-bound GAL1, relative fluorescence intensities have been normalized according to the formula: RFU norm =(RFU/RFU max )*100, where RFU is the relative fluorescence intensity measured and RFU max is the maximal relative fluorescence intensity measured on the array. Isothermal titration calorimetry ITC was used to evaluate the thermodynamics parameters of the binding between GAL1 protein domain and the selected carbohydrates. Purified GAL1 was extensively dialysed in the ITC buffer containing 20 mM phosphate buffer pH 7 or pH 5.2 when the influence on GAL1 carbohydrate binding of either λ5-UR or λ5-UR 22-45 , respectively, was studied. Carbohydrate powders were dissolved directly in the last protein dialysate before experiments. Protein concentration was calculated by measuring the absorbance at 280 nm using a nanodrop ND1000 (Thermoscientific) and titrations were carried out on a MicroCal ITC200 microcalorimeter (GE Healthcare). Each experiment was designed using a titrant concentration (carbohydrate molecule in the syringe) set 10 to 15 times the analyte concentration (protein in the cell) and generally using 17 injections of 2.3 μl at 25 °C (see Supplementary Table 1 for details). A first small injection (generally 0.2 μl) was included in the titration protocol to remove air bubble trapped in the syringe prior titration. λ5-UR or λ5-UR 22-45 peptide was added to the same concentration in both cell and syringe samples for tripartite titration experiments. Integrated raw ITC data were fitted to a one-site non-linear least squares fit model using the MicroCal Origin plugin as implemented in Origin 9.1 (Origin Lab) after the control experiments (titration of the ligand from the syringe into the buffer) were subtracted. Titration experiments performed on GAL1 helped identifying that the protein concentration was generally overestimated in the cell (generally by 20%) due to stability issues. When the associated molar ratio ( N value) could not converge during the fitting process, the N value was set manually and maintained fixed accordingly. Finally, ΔG and TΔS values were calculated from the fitted Δ H and K A values using the equations Δ G =−RTln K A and Δ G =Δ H — T Δ S . NMR spectroscopy The NMR experiments were performed at 303 K on a Bruker Avance III 600 MHz spectrometer equipped with a TCI cryoprobe. The NMR samples contained proteins in 20 mM phosphate buffer pH 5.2. NMR titrations The NMR titrations were performed using 2D 1 H, 15 N HSQC NMR spectra recorded on 15 N-labelled GAL1 (200 μM) in the absence and in the presence of λ5-UR 22-45 peptide (three molar excess). The carbohydrate-binding activity of GAL1 has been determined by recording 2D 1 H, 15 N HSQC spectra of 15 N-labelled GAL1 free or bound to λ5-UR 22-45 after addition of increasing amount of carbohydrate (0.1, 0.2, 0.3, 0.4, 0.8 and 2 mM). The CSPs for each resonance were calculated using the equation: Δ δ obs =[Δ δ HN 2 +(Δ δ N 2 /25)] 1/2 , where Δ δ HN and Δ δ N are, respectively, the proton and nitrogen chemical shifts variation of each residue [51] . STD NMR experiments 1 H and 13 C NMR resonances assignment of LNnT have been performed using 2D 1 H, 13 C HSQC, 2D 1 H, 13 C HSQC-TOCSY, 2D 1 H, 1 H-TOCSY and 2D 1 H, 1 H-COSY experiments. The 1D STD (128 scans, 32 K data points) and the 2D STD TOCSY experiments (mixing time 60 ms with 512 increments of 128 scans each) were performed using a 100:1 LNnT/GAL1 and a 100:1:3 LNnT/GAL1/λ5-UR 22-45 molar ratio samples, with a 1 mM concentration of LNnT. The 1D and 2D STD spectra were recorded with on resonance irradiation at 7.0 p.p.m. and off resonance irradiation at 40 p.p.m. and were performed with a saturation time of 2 s. Cell lines The OP9 and Nalm6 cell lines have been used in the present study since they are able to contact with each other and mediate pre-BCR relocalization [26] . The murine stromal cell line OP9 (ref. 52 ) was cultivated in MEMα, 20% fetal calf serum, 100 U ml −1 penicillin and 100 μg ml −1 streptomycin. The cells were mechanically detached from the dishes using cell scrapers to avoid the use of trypsine. In the OP9 lactose-treated cells, lactose was added to the culture at 0.2 M concentration during 1 h. The human pre-B cell line Nalm6 (ref. 53 ) was cultivated in RPMI, 10% fetal calf serum, 100 U ml −1 penicillin, 100 μg ml −1 streptomycin and 50 μM β-mercaptoethanol. Lectin microarrays All cell samples were prepared and Cy labelled as follows [37] : cells were harvested using a cell scraper and then pelleted (500 g ) and resuspended in PBS. Sonication has been performed and cellular micellae were isolated by means of ultracentrifugation (100,000 g ). We resuspended the pellet in Cy-labelling buffer (0.1 M NaCO 3 in H 2 O, pH 9.3). At this point, we determined the protein concentration by using the DC protein assay (Bio-Rad). We then added at least 10 μg of Cy3- or Cy5- NHS (GE Life Sciences) to 1 mg of cell membrane (as determined by protein content) and incubated for 30 min at room temperature. The labelled cell membrane preps were then dialysed against PBS overnight at 4 °C, aliquoted and snap frozen in liquid N 2 . Aliquots were stored at −80 °C. A reference sample was made by combining equal amounts of OP9 bioreplicated samples into one and labelled. All lectins were purchased from either EY Laboratories (San Mateo, CA) or Vector Laboratories (Burlingame, CA) except TJA-I, TJA-II (NorthStar Bioproducts), cyanovirin (CVN) and scytovirin (SVN; gifts from Dr B. O’Keefe, NCI Frederick). Arrays were printed on Nexterion H slides (SCHOTT North America Inc., Elmsford, NY) using a non-contact printer with piezoelectric dispensing (Nanoplotter 2.1, GeSIM, Germany) at 12 °C and 43% humidity with three spots per lectin per array. Hybridization was performed as previously described [54] . In brief, equal amounts of Cy5-labelled sample was hybridized against Cy3-labelled reference and incubated for 2 h at 25 °C (4 μg total protein brought to a volume of 100 μl with PBS with Tween-20 per array). Lectin activity was monitored using glycoprotein standards to test each array print. Slides were scanned in a GenePix 4300A scanner under normal acquisition mode using GenePix Pro 7.2. The background-subtracted median fluorescence for the three spots per lectin were averaged and log 2 transformed. Signal averages less than 1,000 for both channels were excluded. Lectins with a signal-to-noise ratio <5 for more than 30% of the total data were also excluded. This left 67 of the 107 lectins printed on the array. Each channel was then median normalized per array and the log 2 ratio of sample over reference was calculated. How to cite this article: Bonzi, J. et al . Pre-B cell receptor binding to galectin-1 modifies galectin-1/carbohydrate affinity to modulate specific galectin-1/glycan lattice interactions. Nat. Commun. 6:6194 doi: 10.1038/ncomms7194 (2015).